Mineralized rods and cones suggest colour vision in a 300 Myr-old fossil fish Vision, which consists of an optical system, receptors and image-processing capacity, has existed for at least 520 Myr. Except for the optical system, as in the calcified lenses of trilobite and ostracod arthropods, other parts of the visual system are not usually preserved in the fossil record, because the soft tissue of the eye and the brain decay rapidly after death, such as within 64 days and 11 days, respectively. The Upper Carboniferous Hamilton Formation (300 Myr) in Kansas, USA, yields exceptionally well-preserved animal fossils in an estuarine depositional setting. Here we show that the original colour, shape and putative presence of eumelanin have been preserved in the acanthodii fish Acanthodes bridgei . We also report on the tissues of its eye, which provides the first record of mineralized rods and cones in a fossil and indicates that this 300 Myr-old fish likely possessed colour vision. Evolution of vision in vertebrates is an important theme in the history of animal life. The earliest known purported vertebrate, Myllokunmingia from the Early Cambrian Chengjiang Biota [1] , [2] , [3] , [4] , [5] (~520 Myr), supposedly possessed a rudimentary camera-type eye, but its ultrastructure is unknown. Conodont vertebrates also first appeared in the Cambrian and are presumed to have had large eyes [6] . Except for the optical system, as in the calcified lenses of trilobite and ostracod arthropods, other parts of the visual system are not usually preserved in the fossil record, because the soft tissue of the eye and the brain decay rapidly after death, such as within 64 days and 11 days, respectively [7] . Only five studies have reported a fossilized visual receptor [8] , [9] , [10] , [11] or a mould equivalent [12] , all of which involved arthropod eyes. The lack of receptor preservation in fossilized vertebrate eyes has limited their comparison with the eyes of extant relatives. Opsins are the molecules in extant retinas that are responsible for colour vision. Molecular phylogenetic analyses suggest that four of the five classes of vertebrate opsin genes, and hence colour vision, already existed by the Early Cambrian [13] , [14] . Although colour-producing pigments have been suggested to have been preserved in the external parts of some fossil Mesozoic vertebrates [15] , [16] , [17] , [18] , [19] , [20] , providing some evidence that vertebrates were colour adapted in past geological times, hitherto there has been no direct evidence of colour-sensitive receptors in fossil vertebrates. We here report on the tissues of the eye of the acanthodii fish Acanthodes bridgei , which provides the first record of rods and cones in a fossil and indicates that fish likely possessed colour vision for at least 300 Myr. Morphology of granules Fossils of the acanthodian fish A. bridgei from the Upper Carboniferous Hamilton formation of Kansas show extremely well-preserved skin and articulated cartilages [21] , [22] , [23] . The eyes reveal black and/or dark brown material surrounded by four pieces of sclera skeletal support ( Fig. 1 ). Scanning and transmission electron microscopy (SEM and TEM) confirm observations that many elongate, spindle-shaped granules 1–1.5 μm long ( Fig. 2c,e ) and spherical granules with a diameter <1 μm ( Fig. 2d,f ) occur in the dark brown area of the eye ( Figs 1 and 2a ). The granule area is clearly distinguished from the surrounding limestone matrix area, which has smooth, carbonate crystals ( Supplementary Fig. 1 ). The granules have the same size and shape as the eumelanin granules in the eye of the extant freshwater fish Rhinogobius sp. ( Fig. 2g–j ). 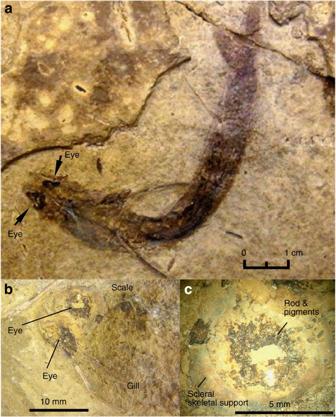Figure 1: Optical photographs of the Carboniferous fishA. bridgei. (a) Complete dorsoventrally compressed specimen (NSM PV22244); the head, including a pair of black/dark brown eyes, is lower left. (b,c) Details of the head region and the right eye (NSM PV22245). Figure 1: Optical photographs of the Carboniferous fish A. bridgei . ( a ) Complete dorsoventrally compressed specimen (NSM PV22244); the head, including a pair of black/dark brown eyes, is lower left. ( b , c ) Details of the head region and the right eye (NSM PV22245). 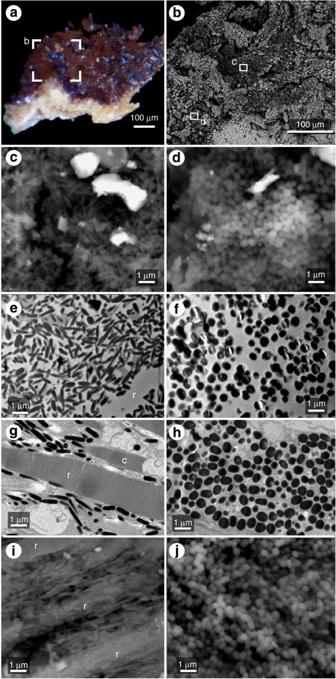Figure 2: Fine structures of the eye of the Carboniferous fishA. bridgeiand extant fishRhinogobiussp. Digital microphotograph (DM), SEM and TEM of an eye ofA. bridgei(a–f, NSM PV22246, 22247), and TEM of the eye ofRhinogobius(g–j, NSM PV22248). (a) DM of a small area of black- and/or brown-coloured eye (NSM PV22246). (b) SEM of the enlarged part ofFig. 2a. (c) SEM of a small region ofbshowing many elongate spindle-shaped granules. (d) SEM of a small region ofbshowing spherical granules found in the lower right area. (e) TEM showing many elongate spindle-shaped granules in the fossilA. bridgei(NSM PV22247). (f) TEM showing many spherical granules in the fossilA. bridgei(NSM PV22247). (g) TEM of the eumelanin found inRhinogobius, between the rod (r) and the cone (c). (h) TEM of retinal pigment epithelium (RPE) melanosomes at the base of the eye in the extantRhinogobius. (i) SEM of eumelanins between the rods (r) inRhinogobius. (j) SEM of RPE melanosomes inRhinogobius. Full size image Figure 2: Fine structures of the eye of the Carboniferous fish A. bridgei and extant fish Rhinogobius sp. Digital microphotograph (DM), SEM and TEM of an eye of A. bridgei ( a – f , NSM PV22246, 22247), and TEM of the eye of Rhinogobius ( g – j , NSM PV22248). ( a ) DM of a small area of black- and/or brown-coloured eye (NSM PV22246). ( b ) SEM of the enlarged part of Fig. 2a . ( c ) SEM of a small region of b showing many elongate spindle-shaped granules. ( d ) SEM of a small region of b showing spherical granules found in the lower right area. ( e ) TEM showing many elongate spindle-shaped granules in the fossil A. bridgei (NSM PV22247). ( f ) TEM showing many spherical granules in the fossil A. bridgei (NSM PV22247). ( g ) TEM of the eumelanin found in Rhinogobius , between the rod (r) and the cone (c). ( h ) TEM of retinal pigment epithelium (RPE) melanosomes at the base of the eye in the extant Rhinogobius . ( i ) SEM of eumelanins between the rods (r) in Rhinogobius . ( j ) SEM of RPE melanosomes in Rhinogobius . Full size image Chemical data The analytical results using alkaline hydrogen peroxide oxidation revealed that high concentrations of pyrrole-2,3,5-tricarboxylic acid (PTCA), pyrrole-2,3-dicarboxylic acid (PDCA) and pyrrole-2,3,4,5-tetracarboxylic acid (PTeCA) occured in the dark brown fragments from the fossil eye, but were absent in the rock matrix ( Table 1 ). These molecules are common only to eumelanin and have never been produced by the alkaline hydrogen peroxide oxidation of any other biological material [24] , [25] , [26] . The PTeCA/PTCA ratio of 2.7 is extremely high as compared with those of extant fish retina (0.10 in Table 1 ) and bovine retinal pigment epithelium melanosomes (0.13), indicating extensive thermal modification of eumelanine [26] , [27] . The retinal area of A. bridgei has many mineralized rods, each about 2 μm wide and maximum length of about 18 μm ( Fig. 3a,c,d ). No immunoreactivity for rhodopsin was observed in the fossil retina ( Supplementary Fig. 2a–d ). On the other hand, the rod-like structures in the retina of living river lizard gobies showed immunoreactivity for rhodopsin ( Supplementary Fig. 2e,f ). These results suggest that rhodopsin, a visual pigment in the visual cells, is not preserved in the fossil retina. Table 1 The analytical results using alkaline hydrogen peroxide oxidation. 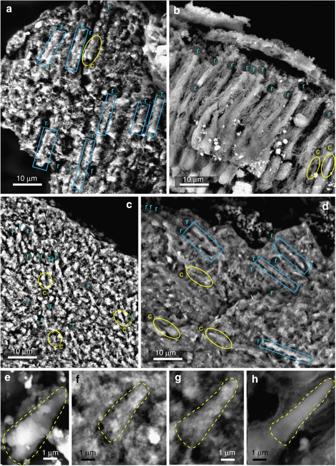Figure 3: SEM and TEM of the rods and cones of the Carboniferous fishA. bridgeiand extant fishRhinogobiussp. A. bridgei(a, NSM PV22249;c–g, NSM PV22250), and SEM and TEM of the eye of the extant fishRhinogobiussp. (b,h). (a–d) SEM of a bundle of rods (r) and cones (c). (e–h) SEM of a cone. Each area of yellow (broken) line and blue (solid) line shows cones and rods, respectively. Full size table Figure 3: SEM and TEM of the rods and cones of the Carboniferous fish A. bridgei and extant fish Rhinogobius sp. A. bridgei ( a , NSM PV22249; c – g , NSM PV22250), and SEM and TEM of the eye of the extant fish Rhinogobius sp. ( b , h ). ( a – d ) SEM of a bundle of rods (r) and cones (c). ( e – h ) SEM of a cone. Each area of yellow (broken) line and blue (solid) line shows cones and rods, respectively. Full size image Morphology of fossil retina Because of the presence of consolidated matrix in the fossil retina, the rods fragmented during the cutting process for TEM observation and so are not well preserved when compared with their counterparts in Rhinogobius sp. The mineralized cones have a basal width of about 2 μm, a height of about 8 μm ( Fig. 3a,c–g ) and their shape, as well as size, is comparable to that of the cones of Rhinogobius sp. ( Fig. 3b,h ). To extract the two principal characters that determine the morphology of the rods and cones, and to determine the distribution of rods and cones within two-dimensional morphospace, principal component analysis (PCA) using elliptic Fourier descriptors was conducted on 509 retinal cells, including the rods and cones of extant vertebrates and A. bridgei . This analysis revealed that the first principal component (PC1) and the third principal component (PC3) account for the relative width of the distal part of retinal cells ( Supplementary Data Sets 1 and 2 ). Extant rods and cones are widely scattered from negative to positive score regions of PC1, although cones tend to be distributed in the more positive score region ( Fig. 4 ). Among 14 photoreceptors of A. bridgei , 8 specimens plotted in the region of cones in extant animals ( Fig. 4 ). Thus, A. bridgei most probably had cones, which suggests that fish have possessed colour vision for at least 300 Myr. 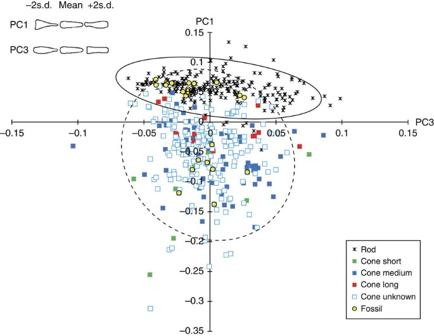Figure 4: Two principal component axes showing the plots for 483 extant vertebrate rod (asterisks) and cone (square) external contours with fossil fish rod and cone contours (yellow). Solid ellipse and dashed ellipse show 95% probability ellipse of extant rods and cones. Upper left column shows theoretical outlines representing variation of the principal components. Figure 4: Two principal component axes showing the plots for 483 extant vertebrate rod (asterisks) and cone (square) external contours with fossil fish rod and cone contours (yellow). Solid ellipse and dashed ellipse show 95% probability ellipse of extant rods and cones. Upper left column shows theoretical outlines representing variation of the principal components. Full size image This is the first discovery of fossil rods and cones in general and, ipso facto , also the first record of receptors, in a fossil vertebrate eye. These findings indicate that such receptors have been conserved in vertebrate eyes for at least 300 Myr. Further, the presence of cones indicates that A. bridgei likely possessed colour vision, although conclusive evidence would require the recovery of opsins. A. bridgei , like Rhinogobius today, inhabited shallow water [22] that would have contained at least most of the wavelengths visible to humans from sunlight. Further, the present study shows that the original colour, shape and putative presence of eumelanin have been conserved for at least 300 Myr, 100 Myr older than previously known [28] . The function of retinal pigment is light absorption [29] . Retinal pigment is contained within the rod and cone cells. However, the retinal pigment epithelium has many functions, such as light absorption, epithelial transport (glucose, vitamin A, Cl − , H 2 O, K + ), 11-cis retinal visual cycle, phagocytosis and secretion (pigment epithelium-derived factor and vascular endothelial growth factor) [29] . The melanin pigment in the retinae of extant vertebrates performs movements that are highly coordinated with the retinomotor movements [30] , [31] , [32] . The existence of rods, cones and melanin pigments in the eye of A. bridgei suggests that retinomotor activity (two modes of vision: daylight vision by cones and crepuscular vision by much more sensitive rods) probably already existed 300 Myr ago. A. bridgei supposedly lived in quite shallow brackish waters [22] . Furthermore, the cone:rod ratios of A. bridgei are comparable with that of extant Rhinogobius ( Fig. 3c,d ), indicating that the fossil fish was diurnal and relied on vision [33] . These results strongly suggest that A. bridgei, the last common ancestor of modern gnathostomes [34] , possessed colour vision, although conclusive evidence would require the recovery of opsins. SEM and TEM observations Fragments of retina levered from the fossil were placed on a stub and viewed under a stereoscopic optical microscope (Nikon SMZ-U) and observed under a SEM (HITACHI TM-1000, TM-3000) uncoated under a low vacuum at the Gunma Museum of Natural History (GMNH) and Japan Agency for Marine-Earth Science and Technology (JAMSTEC). One fragment of retina was fixed overnight in 2% glutaraldehyde with 2% formaldehyde in 0.1 M sodium cacodylate buffer (pH 7.4). The specimen was sent to the Medical School of Okayama University and decalcified with 10% EDTA-2Na (pH 7.4) for ~20 h and post-fixed in 2% osmium tetroxide for ~2.5 h, dehydrated through an ethanol series and embedded in Spurr’s resin and polymerized. Thin sections were obtained using an ultramicrotome, stained with 2% uranyl acetate with 50% ethanol and lead citrate and examined under a TEM (Hitachi H-7650). The living freshwater fish, Rhinogobius sp. (body length 4.5 cm), was selected for comparative purpose because the acanthodian fossil fish is more closely related to actinopterygian fish than to chondrichthyian sharks [35] or the last common ancestor of modern gnathostomes [34] . Furthermore, Rhinogobius lives in quite shallow brackish waters [22] and has a similar body length and eye size to the fossil fish. The specimen was captured using a net basket in a small pond near the GMNH and was fixed using 2.5% glutaraldehyde. Its eyeball was removed and fixed for ~2.5 h, and then cleaved by surgical knife while within the glutaraldehyde solution. The specimen was transferred to the Research Center for Human and Environmental Science of Shinshu University at a temperature of 4 °C. The specimen was rinsed with 0.1 M sodium cacodylate buffer (pH 7.4) and post-fixed in 1% osmium tetroxide for 1 h at 0 °C, then dehydrated through an ethanol series and embedded in Epon resin and polymerized. Thin sections were obtained using an ultramicrotome and then stained with uranyl acetate and lead citrate and examined under a TEM (JEOL JEM-1400HC). Chemical analyses To identify the presence of melanin in the fossil material, the alkaline hydrogen peroxide oxidation method [24] , [25] , [26] , [27] was used in the black to dark brown-coloured fossil eye fragments and the light brown-coloured rock matrix. Samples (8–17 mg) were ground to a fine powder using a mortar and pestle and added to water at a concentration of 10 mg per ml water and 100 μl aliquots were subjected to alkaline hydrogen peroxide oxidation [25] . PTCA and PDCA were analysed by the high-performance liquid chromatography (HPLC) conditions described previously [25] using 0.1 M potassium phosphate buffer (pH 2.1):methanol=99:1, and PTeCA and PTCA were analysed by the HPLC conditions [26] using 0.1 M potassium phosphate buffer (pH 2.1):methanol=88:15. Two separate tests were conducted for fossil eye fragments and rock matrix fragments, respectively. To compare with the fossil fish data, freeze-dried retinal pigment of extant Rhinogobius sp. (0.39 mg) was analysed with the same methods. Morphological analysis of rods and cones Generally speaking, the external contours of the rods and cones have been qualitatively described as rectangular and triangular, respectively. However, the contours of the cones vary from an elongated trapezoid to an equilateral triangle [36] . To describe the contour of the rods and cones quantitatively, an elliptic Fourier analysis was carried out using SHAPE freeware [37] . Images of each rod and cone obtained from the literature ( Supplementary Data Set 1 ; Supplementary Note 1 ) were saved as a RGB bitmap file and converted into a binary image using SHAPE. Subsequently, image noise was manually removed using graphics software (Adobe Photoshop, version 7.01) to obtain an image of only the contour of each rod and cone. The chain-code information ( Supplementary Data Set 2 ) for contour data was normalized and converted to the first 20 harmonics of Fourier coefficients. For the analysis, elliptic Fourier coefficients were normalized for size and alignment of the major axis of the ellipse described by the first harmonic [38] . Because elliptic Fourier analysis yields four coefficients per harmonic, a total of 77 Fourier coefficients were obtained. PCA was used to summarize the coefficients for the 509 retinal cells studied using supplementary software in SHAPE. The PCA was based on the variance–covariance matrix of the coefficients because the primary focus of the present study was variation in gross rod or cone features, rather than fine structure. Geometric interpretation for each principal component was assessed from the reconstructed contours using inverse Fourier transforms. To visualize variation along a principal component axis, inverse Fourier transforms were calculated for mean±2s.d. of the PC scores, with the remaining components set to 0 (ref. 39 ). Immunostaining analysis To examine the preservation of visual pigments in the fossil retina, the specimens were immunostained for rhodopsin, which is a visual pigment of rods. The specimens were thoroughly washed in phosphate buffered saline (PBS, pH 7.4), preincubated by immersion in a blocking solution (PBS containing 5% donkey serum, 0.1% Triton X-100 and 0.05% Tween 20) for 1 h at room temperature, then incubated with a mouse anti-rhodopsin monoclonal antibody (1:500, SMC-176C/D, Stress Marq, Victoria, Canada), which was raised against bovine rhodopsin, overnight at 4 °C in a 96-well plate. After washing in PBS, the specimens were incubated with goat anti-mouse IgG antibody conjugated with Cy3 (1:500, 115-165-003, Jackson, West Grove, PA) together with 4,6-diamidino-2-phenylindole (DAPI, 1:1,000, D9542, Sigma, St. Louis, MO) for 2 h at room temperature. After washing in PBS, the specimens were placed on glass slides, mounted with a medium (Fluoromount, K024, Diagnostic BioSystems, Pleasanton, CA) and coverslipped. For positive control, the retinas of the extant river lizard gobies ( Rhinogobius sp.) were also immunostained for rhodopsin in parallel with the fossil specimens. The gobies were collected from Kamo River in Hiroshima Prefecture, Japan, and kept in tapped water tanks in the laboratory (24 °C) for at least 1 week before use. Because acclimation to darkness is known to facilitate the cleavage of the pigment epithelium layer from the layer of rods and cones in fish retina, the gobies were kept in tap water in dark conditions for at least 1 h and then anaesthetized deeply by adding a 3-ml of tricaine methanesulfonate (50 mg ml −1 , MS-222, E10521, Sigma) into water. The eyeballs were immediately isolated and immersed in 4% paraformaldehyde in 0.1 M phosphate buffer (pH 7.4) for 3 h at 4 °C. The eyeballs were transferred to PBS, then under a binocular stereoscope (SZ61, Olympus, Tokyo, Japan) the pigment epithelium layer was carefully removed by tweezers to expose the layer of rods and cones. The retina was dissected into small pieces (~2 × 2 mm) to obtain the specimen for rhodopsin immunohistochemistry. The specimens were processed using the same procedures as used for immunostaining for rhodopsin in the fossil specimen. Each specimen was examined and photographed under a fluorescent microscope (BX 51, Olympus) equipped with a digital camera (DP 73, Olympus) and analysed using the software ‘cell Sens’ (Olympus). No immunoreactivity was observed in the absence of the primary antibody in control specimens. All the figured specimens were deposited in the National Science Museum, Tokyo (NSM). How to cite this article: Tanaka, G. et al. Mineralized rods and cones suggest colour vision in a 300 Myr-old fossil fish. Nat. Commun. 5:5920 doi: 10.1038/ncomms6920 (2014).